Gating of cyclic nucleotide-gated channels is voltage dependent Cyclic nucleotide-gated channels belong to the family of voltage-gated ion channels, but pore opening requires the presence of intracellular cyclic nucleotides. In the presence of a saturating agonist, cyclic nucleotide-gated channel gating is voltage independent and it is not known why cyclic nucleotide-gated channels are voltage-insensitive despite harbouring the S4-type voltage sensor. Here we report that, in the presence of Li + , Na + and K + , the gating of wild-type cyclic nucleotide-gated A1 and native cyclic nucleotide-gated channels is voltage independent, whereas their gating is highly voltage-dependent in the presence of Rb + , Cs + and organic cations. Mutagenesis experiments show that voltage sensing occurs through a voltage sensor composed of charged/polar residues in the pore and of the S4-type voltage sensor. During evolution, cyclic nucleotide-gated channels lose their voltage-sensing ability when Na + or K + permeate so that the vertebrate photoreceptor cyclic nucleotide-gated channels are open at negative voltages, a necessary condition for phototransduction. Ion channels are membrane proteins that have a fundamental role in neurons and other cell types. They can open in response to voltage and/or ligands (gating), and when open, they allow the passage of specific molecules and ions (permeation) [1] . Since Hodgkin and Huxley's seminal work, permeation and gating have been considered distinct and independent processes [2] , in agreement with recent mutagenesis experiments and crystallographic data [3] , [4] , [5] , [6] , [7] . Ion channels are subdivided into families; the superfamily of voltage-gated channels contains K + , Na + , Ca 2+ , transient receptor potential and cyclic nucleotide-gated (CNG) channels [1] , [8] , [9] , [10] . CNG channels are expressed in vertebrate photoreceptors and olfactory sensory neurons, and mediate sensory transduction [10] , [11] . Native CNG channels are heterotetramers composed of A (CNGA1-A5) and B (CNGB1 and B3) subunits [10] , [11] , [12] . Heterologous expression of CNGA1 channels leads to the formation of functional channels with properties similar, but not identical, to native CNG channels [11] , [12] , [13] , [14] , [15] , [16] . In K + and Na + channels, gating is controlled by 'bundle crossing' at the intracellular side, which controls the opening and closing of the pore [3] , [4] , [5] , [6] . However, in CNG channels, the 'bundle crossing' at the intracellular side does not gate ion permeation; the selectivity filter acts as the gate [10] , [17] . In K + channels, the single-channel open probability ( P o ) increases with the membrane voltage ( V ) because the 'bundle crossing' is removed by the motion of the S4-type voltage sensor, composed of the S1–S4 transmembrane segments [18] . In CNGA1 channels, P o is ~0.85 at positive voltages and ~0.75 at negative voltages in the presence of a saturating agonist concentration (1 mM cGMP) and in the presence of Li + , Na + or K + (refs [19] , [20] , [21] ). Therefore, despite harbouring an S4-type voltage sensor, CNG channels are not thought to be voltage gated. Here, we show that CNG channels are voltage gated in the presence of larger permeating cations. Voltage gating in recombinant WT CNGA1 channels We expressed recombinant wild-type (WT) and CNGA1 mutant channels in Xenopus laevis oocytes and recorded the ionic currents evoked by 1 mM cGMP, a saturating concentration, added to the intracellular side of excised patches under voltage-clamp conditions [22] . The I–V relationship in the presence of 110 mM Li + , Na + or K + on both sides of the membrane was weakly outward rectifying ( Fig. 1a ; Supplementary Fig. S1 ), but in the presence of Rb + or Cs + , the relationship was inward rectifying ( Fig. 1b,c ); the relationship between the relative conductance ( G / G +200 ) and voltage ( V ) depended on the ionic species ( Supplementary Fig. S1 ). Current recordings at −200 mV were noisier than those at +200 mV ( Fig. 1d–g ), and this asymmetry increased with the larger cations Rb + and Cs + . This asymmetry can be quantified by analysing the ratio between the variance of the current σ I 2 and its average value I ; the ratio of σ I 2 / I at −200 mV and at +200 mV |( σ I 2 / I −200 )/( σ I 2 / I +200 )| increased with the ionic radius ( Fig. 1d ) from Na + (1.4) to Cs + (8.5). If CNGA1 channels have a dominant single-channel open state, the ratio σ I 2 / I is equal to i sc (1− P o ), where i sc is the single-channel current, and P o is the open probability (Methods). This ratio is independent of the number of channels present in the membrane patch and is expected to increase when i sc increases and/or P o decreases. The ratio |( σ I 2 / I −200 )/( σ I 2 / I +200 )| is equal to 7.4±1.3 and 8.5±1.4 ( Fig. 1d ) in the presence of symmetrical Rb + and Cs + , respectively, which are far more than the corresponding mean current ratios I −200 / I +200 , equal to 1.57±0.10 and 1.65±0.11, respectively ( Supplementary Fig. S1 ). These observations suggest that for Rb + and Cs + , P o is significantly higher at +200 mV than at −200 mV. If P o is higher at positive voltages than at negative voltages, large tail currents at −200 mV are expected when they are preceded by steps at positive voltages. Indeed, ionic channels that were open at positive voltages will close after a delay when V returns to −200 mV, giving rise to tail currents ( I t ). We measured I t ( V ) at −200 mV evoked by pre-pulses at voltages varying from −100 mV up to +200 mV. In the presence of Na + , I t ( V ) were small ( Fig. 1h ), but I t ( V ) were larger in the presence of Rb + ( Fig. 1i ) and Cs + ( Fig. 1j ). The relationship between the I t / I t_max and V ( Fig. 1k ) obtained from tail currents ( Fig. 1l–n ) is different for Rb + and Cs + . The dependence of the size of I t on the permeating ions is a strong evidence for coupling between gating and permeation. These results suggest the existence of two different voltage-dependent mechanisms operating together in the presence of Rb + and Cs + : an inward rectification of the open pore that reflects asymmetries in ion permeation, and voltage- and time-dependent gating. 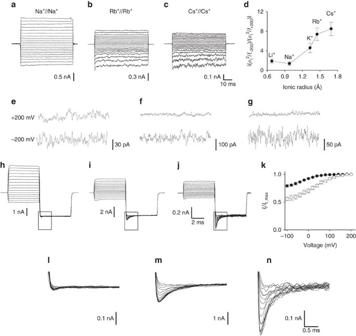Figure 1: Macroscopic currents of recombinant WT CNGA1 channel in symmetrical ionic conditions. (a–c) Macroscopic currents recorded from excised patches in symmetrical solutions of (a) Na+, (b) Rb+and (c) Cs+with 1 mM cGMP on the cytoplasmic side. Voltage steps from −200 to +200 mV (ΔV=20 mV). cGMP-activated currents are outwardly rectifying in Na+, but inwardly rectifying in Rb+and Cs+. (d) Ratios of |(σI2/I−200)/(σI2/I+200)| against ionic radius of alkali cations (n=5 for Li+,n=5 for Na+,n=9 for K+,n=6 for Rb+andn=7 for Cs+). (e–g) Enlargement of macroscopic currents in (e) Na+, (f) Rb+and (g) Cs+, respectively, at ±200 mV. (h–j) Tail currents at −200 mV evoked by pre-pulses at voltages from −100 to +200 mV (ΔV=20 mV); current recordings were filtered at 10 kHz and sampled at 50 kHz to resolve rapid transients. (k) Dependence ofIt/It_maxonVfor Rb+(black circles;n=9) and Cs+(open squares;n=10) from tail currents. (l–n) Enlargement of the tail currents for (l) Na+, (m) Rb+and (n) Cs+, respectively. Data are shown as mean±s.e.m. Figure 1: Macroscopic currents of recombinant WT CNGA1 channel in symmetrical ionic conditions. ( a – c ) Macroscopic currents recorded from excised patches in symmetrical solutions of ( a ) Na + , ( b ) Rb + and ( c ) Cs + with 1 mM cGMP on the cytoplasmic side. Voltage steps from −200 to +200 mV (Δ V =20 mV). cGMP-activated currents are outwardly rectifying in Na + , but inwardly rectifying in Rb + and Cs + . ( d ) Ratios of |( σ I 2 / I −200 )/( σ I 2 / I +200 )| against ionic radius of alkali cations ( n =5 for Li + , n =5 for Na + , n =9 for K + , n =6 for Rb + and n =7 for Cs + ). ( e – g ) Enlargement of macroscopic currents in ( e ) Na + , ( f ) Rb + and ( g ) Cs + , respectively, at ±200 mV. ( h – j ) Tail currents at −200 mV evoked by pre-pulses at voltages from −100 to +200 mV (Δ V =20 mV); current recordings were filtered at 10 kHz and sampled at 50 kHz to resolve rapid transients. ( k ) Dependence of I t / I t_max on V for Rb + (black circles; n =9) and Cs + (open squares; n =10) from tail currents. ( l – n ) Enlargement of the tail currents for ( l ) Na + , ( m ) Rb + and ( n ) Cs + , respectively. Data are shown as mean±s.e.m. Full size image We analysed the properties of single-channel currents in the presence of Rb + and Cs + at −160 and +160 mV ( Fig. 2a,b ). At +160 mV, single-channel currents ( i sc ) had long-lasting openings. Amplitude histograms indicate values for the single-channel conductance ( γ sc ) equal to 5.3±0.5 and 3.9±0.5 pS and P o values of 0.94±0.04 and 0.91±0.05 for the Rb + ( n =6) and Cs + ( n =5) ions, respectively. In contrast, the channel openings were flickery at negative voltages, and the single-channel amplitude could not be measured as precisely as at positive voltages. Channel openings could be estimated from different methods and noise analysis (see Methods) [23] . At −160 mV, the i sc were larger and flickery. The analysis of the amplitude histograms revealed the existence of two open states for Rb + ( n =6) with γ sc equal to 8.6±0.7 and 14.6±0.9 pS ( Fig. 2a ). In the presence of Cs + , i sc had amplitudes up to 5 pA, whereas no well-resolved open state could be detected from the all-point histogram, and the single-channel amplitude measured from peak analysis ( i sc_p ) was 2.3 pA ( Fig. 2b ). At −160 mV, γ sc_p for Cs + was 13.4±2.5 pS, and P o was 0.65±0.06 and 0.27±0.07 for Rb + ( n =5) and Cs + ( n =4), respectively. Flickering openings at negative voltages in the presence of Cs + are unlikely to be caused by a cationic blockage, as flickering blockage is associated with a decrease of i sc , in contrast with what was observed. In Rb + and Cs + , both γ sc and P o depend on V but in an opposite way; γ sc decreases, but P o increases from −160 to +160 mV ( Fig. 2c–f ). The opposite effect of V on γ sc and P o covers a voltage-dependent gating, which can be inferred by the analysis of current fluctuations and properly observed only in single-channel recordings. The dependence of γ sc and P o on V reveals the existence of a voltage sensor in CNGA1 channels, that is, a molecular structure sensing changes in the electric field and transducing it into a conformational change [18] . If this voltage sensor becomes effective when Rb + and Cs + permeate ( Fig. 1 ), it could be located in the pore itself and be distinct from the S4-type voltage sensor of K + channels. 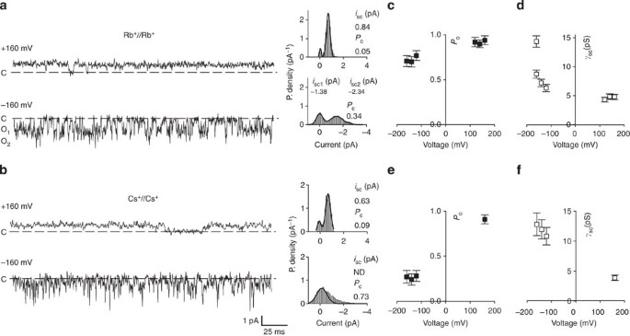Figure 2: Single-channel currents of recombinant WT CNGA1 channel in symmetrical ionic conditions. (a) Current recordings at +160 mV and −160 mV from the same single WT CNGA1 channel in the presence of 1 mM cGMP in symmetrical Rb+; current recordings were filtered at 5 kHz and sampled at 20 kHz. Dashed lines in single-channel recordings indicate the closed state (C) of the channel; O1and O2indicate the open state levels. All-point histograms are shown at the right of each trace.iscandPcindicate the single-channel current and the closed probability, respectively. (b) The same as inabut for Cs+. ND, not determined. (c) Dependence of open probability (Po) onVfor symmetrical Rb+(filled squares;n=6). (d) Dependence of single-channel conductance (γsc) onVfor symmetrical Rb+(open squares;n=6). (e) The same as incbut for Cs+(n=5). (f) The same as indbut for Cs+(n=5).Powas estimated as 1−Pcfrom normalized all-point histograms. Data are shown as mean±s.e.m. P. density, probability density. Figure 2: Single-channel currents of recombinant WT CNGA1 channel in symmetrical ionic conditions. ( a ) Current recordings at +160 mV and −160 mV from the same single WT CNGA1 channel in the presence of 1 mM cGMP in symmetrical Rb + ; current recordings were filtered at 5 kHz and sampled at 20 kHz. Dashed lines in single-channel recordings indicate the closed state (C) of the channel; O 1 and O 2 indicate the open state levels. All-point histograms are shown at the right of each trace. i sc and P c indicate the single-channel current and the closed probability, respectively. ( b ) The same as in a but for Cs + . ND, not determined. ( c ) Dependence of open probability ( P o ) on V for symmetrical Rb + (filled squares; n =6). ( d ) Dependence of single-channel conductance ( γ sc ) on V for symmetrical Rb + (open squares; n =6). ( e ) The same as in c but for Cs + ( n =5). ( f ) The same as in d but for Cs + ( n =5). P o was estimated as 1− P c from normalized all-point histograms. Data are shown as mean±s.e.m. P. density, probability density. Full size image The voltage sensor inside the pore CNG and K + channels have a significant sequence identity in the pore region (23%) and are thought to share a similar three-dimensional structure [10] , [11] , [24] . In the filter region of K + channels, there is a signature formed by the amino acids T(V/I)GYG, while in CNG channels, an ETPP motif follows after the conserved TIG residues ( Fig. 3a ). The recently determined crystal structures of the CNG-mimicking NaK chimeras [25] are good templates for the pore region of CNG channels. These chimeras were obtained from the NaK channel template by reproducing the CNG selectivity filter sequence in the NaK channel [25] background ( Fig. 3a ). The pore region of CNGA1 channels is formed by the residues T (359) TIGET (364) ( Fig. 3a ), and the crystal structure of the pore based on the NaK2CNG-E [25] chimera ( Fig. 3b ) suggests that the side chain of Thr360 points towards the pore axis, while the side chains of Thr364, Glu363, Iso361 and Thr359 point away from the ion conduction pathway. Residues Thr359, Thr360, Iso361, Glu363 and Thr364 in CNGA1 correspond to Thr62, Thr63, Iso64, Glu66 and Thr67, respectively, in the NaK2CNG-E chimera ( Fig. 3a,b ). The only charged residue in the pore is Glu363, and it could be part of a pore voltage sensor. Therefore, we investigated mutant channel E363A known to desensitize [26] , [27] , that is, the current in the presence of a steady concentration of cGMP declines with a time constant of 5–10 s at positive voltages and more rapidly at negative voltages ( Supplementary Fig. S2 ). When the cGMP-activated current has declined to its steady level, it is possible to compare current fluctuations obtained for similar values of the macroscopic current I at positive and negative V by using the appropriate cGMP concentrations. In symmetrical Na + ( Fig. 4a ), Rb + ( Fig. 4b ) and Cs + ( Fig. 4c ), fluctuations at ±200 mV had approximately the same amplitude (compared with the corresponding data in the WT CNGA1 channels in Fig. 1 ). In contrast with WT CNGA1 channels, the ratio |( σ I 2 / I −200 )/( σ I 2 / I +200 )| in mutant channels E363A did not increase with the ionic radius ( Fig. 4d ). Stationary fluctuation analysis of macroscopic currents in Rb + ( Fig. 4e ) and Cs + ( Fig. 4f ) at low cGMP concentrations indicated similar values for i sc at ±160 mV. Moreover, brief transient currents were recorded from the membrane patches containing a few or possibly only one channel, showing very similar amplitudes at ±160 mV ( Fig. 4g,h ; Supplementary Fig. S3 ). Fluctuation measurements of macroscopic currents ( Fig. 4 ) and the peak analysis of the brief transient current indicate that in mutant channels E363A, the voltage dependency of γ sc in the presence of Rb + or Cs + is drastically reduced. Very similar results were observed in mutant channels T364A ( Supplementary Figs S2,S3 ). We have also performed titration experiments in WT channels, by varying the extracellular pH inside the patch pipette while keeping the intracellular pH constant ( Supplementary Fig. S4 ). Lowering the extracellular pH results in a reversible voltage- and time-dependent desensitisation ( Supplementary Fig. S4 ), similar to that of the E363A mutant channel ( Supplementary Fig. S2 ) and in a progressive, outward rectification ( Supplementary Fig. S5 ). This result provides further evidence for the existence of the interactions of the carboxyl group of Glu363 with other residues in the pore. These observations suggest the existence of a voltage sensor in the pore of WT CNGA1 channels, in which the carboxyl groups of Glu363 and the polar groups of Thr364 are essential components. 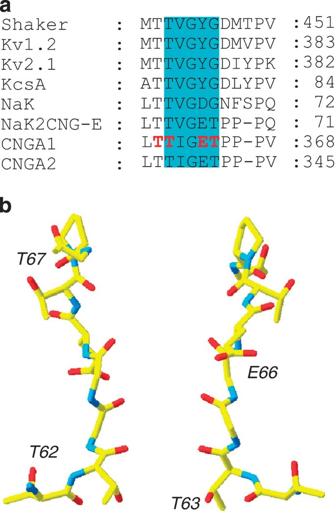Figure 3: Sequence alignment in the selectivity filter for different ion channels and molecular structure of the CNG-mimicking NaK chimera. (a) Sequence alignment of the selectivity filter of Shaker (GI, 13432103), Kv1.2 (GI, 25742772), Kv2.1 (GI, 6981120), KcsA (GI, 61226909), NaK (GI, 218766679), NaK2CNG-E (GI, 317455146), CNGA1 (GI, 296486581) and CNGA2 (GI, 296471151) channels. The TVGYG signature of K+channels is highlighted in blue; in red, mutated residues of the CNGA1 channel. (b) Partial molecular structure of the mimics of the CNGA1 channel obtained from the NaK2CNG-E crystal structure25as deposited in the Protein Data Bank (PDB accession code3K0D) featuring the selectivity filter in two diagonally opposite subunits. Figure 3: Sequence alignment in the selectivity filter for different ion channels and molecular structure of the CNG-mimicking NaK chimera. ( a ) Sequence alignment of the selectivity filter of Shaker (GI, 13432103), Kv1.2 (GI, 25742772), Kv2.1 (GI, 6981120), KcsA (GI, 61226909), NaK (GI, 218766679), NaK2CNG-E (GI, 317455146), CNGA1 (GI, 296486581) and CNGA2 (GI, 296471151) channels. The TVGYG signature of K + channels is highlighted in blue; in red, mutated residues of the CNGA1 channel. ( b ) Partial molecular structure of the mimics of the CNGA1 channel obtained from the NaK2CNG-E crystal structure [25] as deposited in the Protein Data Bank (PDB accession code 3K0D ) featuring the selectivity filter in two diagonally opposite subunits. 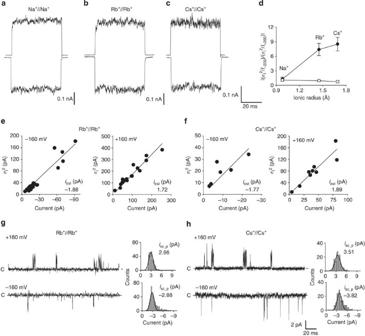Figure 4: Macroscopic and single-channel properties in the E363A mutant channels. (a–c) Comparison between fluctuations of macroscopic currents of a similar amplitude activated by different cGMP concentrations (50 μM–1 mM) in mutant channels E363A at ±200 mV in the presence of (a) Na+, (b) Rb+and (c) Cs+. (d) Ratios of |(σI2/I−200)/(σI2/I+200)| against ionic radius of alkali cations for E363A (open circles;n≥4) and WT (black circles;n≥5). (e) Stationary fluctuation analysis at −160 mV (left panel) and +160 mV (right panel) in symmetrical Rb+. (f) As inebut for Cs+. The experimental relation betweenσI2andIfor (e) Rb+and (f) Cs+obtained at low cGMP concentration (50 μM) shows a similar slope at positive and negative voltages providing an estimate of single-channel current amplitude (iest). (g,h) E363A single-channel currents in symmetrical (g) Rb+and (h) Cs+at −160 mV and +160 mV in the presence of 1 mM cGMP. Dashed lines in single-channel recordings indicate the closed state (C) of the channel. Amplitude histograms are shown at the right of each trace.isc_pindicates the estimated single-channel current amplitude. Data are shown as mean±s.e.m. Full size image Figure 4: Macroscopic and single-channel properties in the E363A mutant channels. ( a – c ) Comparison between fluctuations of macroscopic currents of a similar amplitude activated by different cGMP concentrations (50 μM–1 mM) in mutant channels E363A at ±200 mV in the presence of ( a ) Na + , ( b ) Rb + and ( c ) Cs + . ( d ) Ratios of |( σ I 2 / I −200 )/( σ I 2 / I +200 )| against ionic radius of alkali cations for E363A (open circles; n ≥4) and WT (black circles; n ≥5). ( e ) Stationary fluctuation analysis at −160 mV (left panel) and +160 mV (right panel) in symmetrical Rb + . ( f ) As in e but for Cs + . The experimental relation between σ I 2 and I for ( e ) Rb + and ( f ) Cs + obtained at low cGMP concentration (50 μM) shows a similar slope at positive and negative voltages providing an estimate of single-channel current amplitude ( i est ). ( g , h ) E363A single-channel currents in symmetrical ( g ) Rb + and ( h ) Cs + at −160 mV and +160 mV in the presence of 1 mM cGMP. Dashed lines in single-channel recordings indicate the closed state (C) of the channel. Amplitude histograms are shown at the right of each trace. i sc_p indicates the estimated single-channel current amplitude. Data are shown as mean±s.e.m. Full size image In the pore there are two additional polar residues, Thr360 and Thr359 ( Fig. 3a ), which could be part of the pore voltage sensor. Mutant channels T360A and T359A do not desensitize [26] , and their macroscopic currents do not exhibit any outward or inward rectification in the presence of symmetrical Na + ( Fig. 5a,h ), Rb + ( Fig. 5b,i ) or Cs + ( Fig. 5c,j ). However, a closer analysis of current fluctuations reveals an altered gating ( Fig. 5e–g and l–n ); indeed, in both mutant channels T359A and T360A, the ratios |( σ I 2 / I −200 )/( σ I 2 / I +200 )| in the presence of symmetrical Na + were 3.1 and 2.7, respectively, which is slightly higher than 1.4 observed in WT CNGA1 channels. In the presence of symmetrical Cs + , the ratios were 4.9 and 3.2, respectively, which is significantly less than the value of 8.5 measured in the WT CNGA1 channels ( Fig. 5d,k ). In contrast, this ratio was larger than 10 in the presence of symmetrical Rb + , suggesting different single-channel properties at positive and negative voltages ( Fig. 5d,f,k,m ). In mutant channels T359A and T360A in the presence of symmetrical Rb + , the single-channel properties at positive and negative voltages were more different than in WT CNGA1 channels ( Fig. 2 ). At +160 mV, long-lasting openings were observed with a P o of 0.95±0.03 and a γ sc of 30 pS ( n =3), while at −160 mV, two open states were observed. One state had a γ sc equal to 15.8±1.2 pS with a P o equal to 0.83±0.03, and the other state was more flickering with a P o equal to 0.12±0.02 ( n =4) with variable openings up to 20 pA ( Fig. 5o ). In contrast, single-channel openings had similar properties at positive and negative voltages in symmetrical Cs + ( Fig. 5p ), but the open channel noise had a variance 1.8 times larger at negative voltages, suggesting that the channels undergo rapid, unresolved transitions more frequently at these voltages [28] . In symmetrical Cs + , the mutant channel T359A showed P o values of 0.95±0.03 ( n =3) and 0.91±0.03 ( n =3) at +160 and −160 mV, respectively, and the i sc values were 1.2±0.2 ( n =3) and 1.0±0.3 ( n =3) at +160 and −160 mV, respectively. These results show that Glu363 and Thr364 contribute to the voltage dependence of γ sc during Rb + and Cs + permeation, and suggest that they could operate in a coordinated fashion. The polar Thr359 and Thr360 residues at the intracellular entrance appear to modulate the effect of the permeating ion on gating. 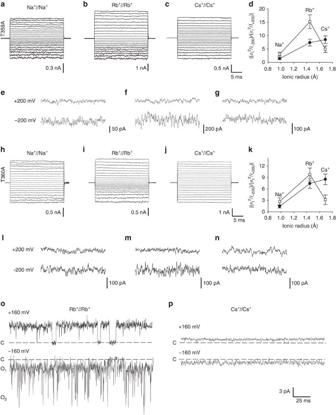Figure 5: Macrcoscopic and single-channel currents recordings in T359A and T360A mutant channels in symmetrical ionic conditions. (a–c) Macroscopic currents recorded in T359A pore mutant channel from excised patches in symmetrical solutions of (a) Na+, (b) Rb+and (c) Cs+. Experimental protocols were as described inFig. 1. (d) Ratios of |(σI2/I−200)/(σI2/I+200)| against ionic radius of alkali cations for T359A mutant channels (open squares;n≥5) and WT CNGA1 (black circles;n≥5). (e–g) Enlargement of macroscopic current in (e) Na+, (f) Rb+and (g) Cs+, respectively, at ±200 mV. (h–j) Macroscopic currents recorded in T360A pore mutant channels in symmetrical solutions of (h) Na+, (i) Rb+and (j) Cs+. (k) Ratios of |(σI2/I−200)/(σI2/I+200)| against ionic radius of alkali cations for T360A mutant channels (open squares;n≥4) and WT CNGA1 (black circles;n≥5). (l–n) Enlargement of macroscopic current in (l) Na+, (m) Rb+and (n) Cs+, respectively, at ±200 mV. (o,p) T359A single-channel currents in symmetrical (o) Rb+and (p) Cs+at −160 and +160 mV in the presence of 1 mM cGMP. Current recordings were filtered at 5 kHz and sampled at 10 kHz. Dashed lines in single-channel recordings indicate the closed state (C) of the channel; O1and O2indicate the open state levels. Data are shown as mean±s.e.m. Figure 5: Macrcoscopic and single-channel currents recordings in T359A and T360A mutant channels in symmetrical ionic conditions. ( a – c ) Macroscopic currents recorded in T359A pore mutant channel from excised patches in symmetrical solutions of ( a ) Na + , ( b ) Rb + and ( c ) Cs + . Experimental protocols were as described in Fig. 1 . ( d ) Ratios of |( σ I 2 / I −200 )/( σ I 2 / I +200 )| against ionic radius of alkali cations for T359A mutant channels (open squares; n ≥5) and WT CNGA1 (black circles; n ≥5). ( e – g ) Enlargement of macroscopic current in ( e ) Na + , ( f ) Rb + and ( g ) Cs + , respectively, at ±200 mV. ( h – j ) Macroscopic currents recorded in T360A pore mutant channels in symmetrical solutions of ( h ) Na + , ( i ) Rb + and ( j ) Cs + . ( k ) Ratios of |( σ I 2 / I −200 )/( σ I 2 / I +200 )| against ionic radius of alkali cations for T360A mutant channels (open squares; n ≥4) and WT CNGA1 (black circles; n ≥5). ( l – n ) Enlargement of macroscopic current in ( l ) Na + , ( m ) Rb + and ( n ) Cs + , respectively, at ±200 mV. ( o , p ) T359A single-channel currents in symmetrical ( o ) Rb + and ( p ) Cs + at −160 and +160 mV in the presence of 1 mM cGMP. Current recordings were filtered at 5 kHz and sampled at 10 kHz. Dashed lines in single-channel recordings indicate the closed state (C) of the channel; O 1 and O 2 indicate the open state levels. Data are shown as mean±s.e.m. Full size image The role of S4 in voltage gating The high amino-acid conservation (30% identity and 75% similarity) in the S4 segment between CNGA1 and Kv1.2. channels ( Fig. 6a ) and the observation that the paddle motif (S3b-S4) from CNGA1 channels sustains voltage-dependent gating in a chimeric Shaker channel [29] raise an obvious question: does the S4 segment contribute to voltage gating in the presence of Rb + and Cs + ? The first four positive charges in S4 are highly conserved among the K + , Na + and Ca 2+ channels [6] , [7] , [18] and correspond to Arg269, Arg272, Arg275 and Arg278 (here referred to as R1, R2, R3 and R4) in CNGA1 channels. Therefore, we investigated whether their neutralisation alters gating. When the messenger RNA coding for mutant channels R1Q, R2Q, R3Q, R4Q, R1T, R2T and R3T was injected into oocytes, cGMP-activated currents were either too small to be observed or absent (data not shown). cGMP-activated currents, however, were recorded in mutant channels R4T and in the tandem constructs R1Q_WT and R2Q_WT, that is, constructs where the mutant channel (R1Q or R2Q) was attached by an appropriate linker to a WT CNGA1 subunit ( Fig. 6b–g ). No cGMP-activated currents were recorded from the R3Q_WT tandem. Current recordings in the presence of symmetrical Rb + and Cs + for R1Q_WT and R4 T mutant channels ( Fig. 6b,c,f,g ) have the same rectification and kinetics of WT CNGA1 channels. In the tandem construct R2Q_WT, the inward rectification observed in the presence of Rb + in the WT CNGA1 channel was less pronounced ( Fig. 6d,h ). For Cs + , macroscopic currents of R2Q_WT channels ( Fig. 6e ) did not show the inward rectification observed in the WT CNGA1 channels ( Fig. 6i ). 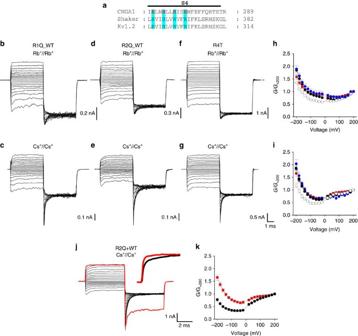Figure 6: R2Q mutant channels in S4 transmembrane domain. (a) Sequence alignment between CNGA1, Shaker and Kv1.2 in the S4 domain. Arginines (R) are highlighted in blue; mutated residues in red. (b,c) Tail currents at −200 mV evoked by pre-pulses at voltages from −180 to +200 mV (ΔV=20 mV) in symmetrical (b) Rb+and (c) Cs+for R1Q_WT tandem construct. (d,e) The same as inbandcbut for tandem construct R2Q_WT. (f,g) The same as inbandcbut for mutant channel R4T. (h,i) Dependence ofG/G+200onVin (h) Rb+and (i) Cs+for WT (red squares;n≥9), R1Q_WT (black circles;n≥5), R2Q_WT (open circles;n≥5) and R4T (blue circles;n≥4). (j) Tail currents at −200 mV for co-injected R2Q+WT mutant channels evoked by pre-pulses from −180 to +200 mV. Normalized WT CNGA1 current (in red) evoked by pre-pulse at +200 mV is superimposed; the inset shows an enlargement of initial parts of normalized current traces at +200 mV in Cs+for mutant (in black) and WT CNGA1 channels (in red). Current recordings were filtered at 10 kHz and sampled at 50 kHz. (k) Dependence ofG/G+200onVin Cs+for R2Q+WT (black circles;n=5) and WT CNGA1 channels (red squares;n=10). Data are shown as mean±s.e.m. Figure 6: R2Q mutant channels in S4 transmembrane domain. ( a ) Sequence alignment between CNGA1, Shaker and Kv1.2 in the S4 domain. Arginines (R) are highlighted in blue; mutated residues in red. ( b , c ) Tail currents at −200 mV evoked by pre-pulses at voltages from −180 to +200 mV (Δ V =20 mV) in symmetrical ( b ) Rb + and ( c ) Cs + for R1Q_WT tandem construct. ( d , e ) The same as in b and c but for tandem construct R2Q_WT. ( f , g ) The same as in b and c but for mutant channel R4T. ( h , i ) Dependence of G / G +200 on V in ( h ) Rb + and ( i ) Cs + for WT (red squares; n ≥9), R1Q_WT (black circles; n ≥5), R2Q_WT (open circles; n ≥5) and R4T (blue circles; n ≥4). ( j ) Tail currents at −200 mV for co-injected R2Q+WT mutant channels evoked by pre-pulses from −180 to +200 mV. Normalized WT CNGA1 current (in red) evoked by pre-pulse at +200 mV is superimposed; the inset shows an enlargement of initial parts of normalized current traces at +200 mV in Cs + for mutant (in black) and WT CNGA1 channels (in red). Current recordings were filtered at 10 kHz and sampled at 50 kHz. ( k ) Dependence of G / G +200 on V in Cs + for R2Q+WT (black circles; n =5) and WT CNGA1 channels (red squares; n =10). Data are shown as mean±s.e.m. Full size image In the tandem construct R2Q_WT, the amino terminus of the voltage sensor, composed of the S1–S4 transmembrane segments, is linked to the carboxy terminus of the other subunit of the tandem; this linker could perturb the physiological operation of the voltage sensor. Indeed, the C-termini of three subunits of WT CNGA1 could be linked together by a parallel three-helix coiled-coil domain of a leucine zipper region [30] , and this trimeric structure could be distorted or destroyed in channels formed by two tandems in which one C-terminus is linked to the N-terminus of another subunit. Therefore, we investigated the properties of ion channels obtained when the mutant channels R1Q, R2Q and R3Q were co-expressed in a 1:1 ratio with WT CNGA1 channels (hereafter referred to as R1Q+WT, R2Q+WT and R3Q+WT), where the C-termini are free to form leucine zippers. In the presence of symmetrical Na + and Rb + , cGMP-activated currents in the mutant channels R1Q+WT, R2Q+WT and R3Q+WT were very similar to those recorded in the WT CNGA1 channels ( Supplementary Fig. S6 ). In contrast, the macroscopic currents of the R2Q+WT channels were outwardly rectifying in the presence of Cs + ( Fig. 6j,k ). The effect of neutralisation of R2 in the S4 domain was better seen when cGMP-activated currents, obtained with voltage steps from 0 to +200 and then to −200 mV, in WT CNGA1 channels were normalized to the maximal current recorded at +200 mV in R2Q+WT channels (red trace in Fig. 6j ). When V was stepped from 0 to +200 mV, cGMP-activated currents in the R2Q+WT mutant channels reached their maximum amplitude with a delay of 0.5–1 ms compared with the WT CNGA1 channels (inset in Fig. 6j ), but the peak of the tail currents observed when the voltage was stepped to – 200 mV was very similar in the R2Q+WT and WT CNGA1 channels. The longer delay with which the cGMP-activated current reached its peak when R2 was neutralized suggests that S4 moves through a more shallow energy landscape, consistent with the notion that fewer gating charges cross the electric field of the membrane [18] . The relationship between G / G +200 and V in symmetrical Cs + shows that the rectification observed in WT CNGA1 channels is inverted in R2Q+WT channels ( Fig. 6j,k ). The similarity of the results obtained with the tandem construct R2Q_WT and with the coinjection of mutant R2Q and WT CNGA1 channels strongly suggests that the altered gating observed in the tandem construct R2Q_WT is not due to the linker inserted between the N and C termini of different subunits but that it is indeed caused by the neutralisation of Arg272 in the S4 domain. Voltage gating of organic cations In the mutant channels R2Q_WT and R2Q+WT, the voltage gating of Rb + is very similar to that observed in WT CNGA1 channels, but not for Cs + ( Fig. 6 ). This observation suggests that the size of the permeating ion is important, raising the possibility that S4 is primarily involved in the voltage gating of large ions and not that of small ions such as Li + , Na + and K + . Therefore, we examined gating in the presence of larger organic cations such as methylammonium (MA; 3.5×3.7×4.1 Å) and dimethylammonium (DMA; 3.8×4.2×6.1 Å). In MA and DMA, which cannot form hydrogen bonds, the I/V relationship was outward rectifying ( Fig. 7a–c ), and the ratio | I +200 / I −200 | was 2.9±0.4 and 7.6±0.8 for MA ( n =6) and DMA ( n =5), respectively ( Fig. 7a–c ). Single-channel recordings from these channels confirm that the voltage-dependent activation is caused by channel gating rather than a voltage-dependent change of γ sc ( Supplementary Fig. S7a ). The outward rectification observed in the presence of MA was enhanced in the R2Q_WT tandem and became 6.1±0.4 ( n =3) for MA ( Fig. 7d,e ). Very similar results were obtained in the mutant R2Q+WT channels ( Supplementary Fig. S7b ). The outward rectification observed in the presence of MA and DMA could be caused by an open-pore blockage from these organic cations binding to a site in the intracellular vestibule [31] . To exclude this possibility, we investigated the fractional block of the Na + inward current by intracellular MA and DMA at very negative voltages. Under these experimental conditions, when MA or DMA is in the bathing medium and Na + ions in the patch pipette, the open-pore block by MA and DMA is progressively relieved at negative voltages and is almost absent at −200 mV ( Supplementary Fig. S8 ). 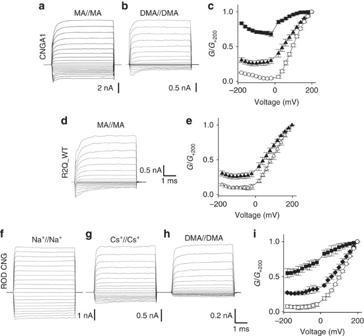Figure 7: Permeation of large organic cations in recombinant and native CNG channels. (a,b) Macroscopic currents in symmetrical solutions (110 mM) of (a) MA and (b) DMA for WT CNGA1 channels. (c) Dependence ofG/G+200onVfor Na+(black squares;n=7), MA (black triangles;n=6) and DMA (open circles;n=5) for WT CNGA1 channels. (d) Macroscopic current in symmetrical MA for R2Q_WT construct. (e) Dependence ofG/G+200onVfor MA in WT CNGA1 (black triangles;n=6) and R2Q_WT channels (open triangles;n=4). (f–h) Macroscopic currents in symmetrical solutions (110 mM) of (f) Na+, (g) Cs+and (h) DMA from native rod CNG channels. (i) Dependence ofG/G+200onVfor Na+(filled squares;n=4), Cs+(filled diamonds;n=4) and DMA (open circles;n=3) for native rod CNG channels. Current recordings were filtered at 5 kHz and sampled at 20 kHz. Data are shown as mean±s.e.m. Figure 7: Permeation of large organic cations in recombinant and native CNG channels. ( a,b ) Macroscopic currents in symmetrical solutions (110 mM) of ( a ) MA and ( b ) DMA for WT CNGA1 channels. ( c ) Dependence of G / G +200 on V for Na + (black squares; n =7), MA (black triangles; n =6) and DMA (open circles; n =5) for WT CNGA1 channels. ( d ) Macroscopic current in symmetrical MA for R2Q_WT construct. ( e ) Dependence of G / G +200 on V for MA in WT CNGA1 (black triangles; n =6) and R2Q_WT channels (open triangles; n =4). ( f – h ) Macroscopic currents in symmetrical solutions (110 mM) of ( f ) Na + , ( g ) Cs + and ( h ) DMA from native rod CNG channels. ( i ) Dependence of G / G +200 on V for Na + (filled squares; n =4), Cs + (filled diamonds; n =4) and DMA (open circles; n =3) for native rod CNG channels. Current recordings were filtered at 5 kHz and sampled at 20 kHz. Data are shown as mean±s.e.m. Full size image A very similar voltage-dependent gating was observed in native CNG channels from newt rod outer segments. In symmetrical Na + , Cs + and DMA, the cGMP-activated current was progressively more outward rectifying ( Fig. 7f–i ), and in DMA the ratio of | I +200 / I −200 | was larger than 10 ( Fig. 7h,i ). The strong correlation between the dimension of the permeating ions and the degree of the voltage dependency suggests that similar mechanisms to those described for recombinant WT CNGA1 channels operate in native CNG channels from rods. In the present article, we show that CNG channels display weak voltage gating for the three smallest alkali monovalent cations (Li + , Na + and K + ), whereas their gating is voltage dependent for larger cations, such as Rb + , Cs + , MA and DMA. Gating and permeation in CNGA1 channels are strongly coupled [32] , [33] , [34] , and we show that this coupling is modulated by the voltage acting on specific charged protein structures: a pore voltage sensor and the S4-type voltage sensor. We propose that the charged Glu363 and polar Thr364 at the extracellular entrance of the selectivity filter determine the coupling between gating and permeation and, in particular, the asymmetry of the single-channel conductance at positive and negative voltages, while the polar Thr359 and Thr360 at the intracellular entrance modulate the action of the permeating ion. In voltage-gated channels, the relationship I t / I t_max is often used to infer the dependence of P o / P o_max on V from the macroscopic currents. In the presence of symmetrical Rb + , the P o / P o_max in WT CNGA1, R2Q_WT and R2Q+WT channels is very similar ( Fig. 8a ). In contrast, the WT CNGA1 channel P o / P o_max reaches a clear plateau around +180 mV in the presence of symmetrical Cs + , which is not the case when Arg272 is neutralized. In fact, in the mutant channels R2Q_WT and R2Q+WT, the P o / P o_max is shifted towards more positive voltages ( Fig. 8b ). The dependence of P o / P o_max on V is fitted with a Boltzmann equation plus a pedestal (see Methods), helping to elucidate the mechanisms underlying the observed voltage-dependent gating. First, when Arg272 is neutralized in symmetrical Cs + and MA, the activation midpoint ( V 1/2 ) shifts towards more positive voltages, suggesting the involvement of the S4-type voltage sensor in voltage gating, as observed in voltage-gated K + channels [35] , [36] , [37] and transient receptor potential channels [38] after neutralisation of charged residues in S4. Second, the small value of the effective charge ( z ), equal to 0.74±0.03, 0.52±0.02 and 0.51±0.02 for Rb + , Cs + and MA, respectively, is consistent with the limited motion of charges during voltage gating in WT CNGA1 channels, significantly less prominent than that in voltage-gated K + channels, where the value of z ranges from 2 to 4 (refs [29] , [35] , [36] , [37] ). 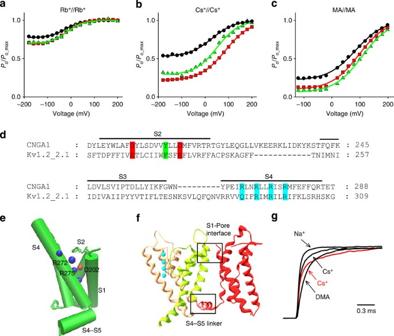Figure 8: Voltage-dependent gating in WT CNGA1 channels and possible underlying molecular mechanisms. (a) Dependence ofPo/Po_maxonVfor Rb+from tail currents in WT (black circles), R2Q+WT (red squares) and R2Q_WT (green triangles) channels. Data were fitted with a Boltzmann function as described in the Methods with C,V1/2andzequal to: 0.77±0.01, 21.6±1.6 and 0.74±0.03 for WT; 0.69±0.01, 17.1±1.6 and 0.72±0.03 for R2Q+WT mutant; 0.70±0.01, 16.4±4.6 and 0.73±0.08 for R2Q_WT mutant channels.It/It_maxis an estimation ofPo/Po_max. (b) The same as inabut for Cs+. C,V1/2andzare as follow: 0.53±0.01, 29.5±1.9 and 0.52±0.02 for WT; 0.21±0.01, 87.1±0.9 and 0.47±0.01 for R2Q+WT mutant; 0.29±0.01, 50.8±3.1 and 0.54±0.03 for R2Q_WT mutant channels. (c) Dependence ofPo/Po_maxonVin MA for the same mutant channels as ina. C,V1/2andzare as follow: 0.21±0.01, 83.6±1.7 and 0.51±0.02 for WT; 0.09±0.02, 94.9±1.6 and 0.52±0.02 for R2Q+WT mutant; 0.06±0.01, 106.1±1.8 and 0.51±0.02 for R2Q_WT mutant channels. (d) Sequence alignment between the voltage sensor of CNGA1 and the Kv1.2–Kv2.1 chimera. Arginine residues (R) in S4 are highlighted in blue. Highly conserved negatively charged residues in S2 forming the external negative cluster (E214) and internal negative cluster (E224) are shown in red. (e) A cartoon of CNGA1 voltage sensor based on the crystal structure of Kv1.2–2.1 (PDB ID 2R9R) where the negative aspartate in position 202 could be involved in a salt bridge with Arg272 stabilizing the activated state of the voltage sensor is shown. (f) Cartoon of a monomeric subunit of chimera Kv1.2–Kv2.1 and the pore region from the adjacent subunit showing two possible interfaces (indicated by the squares) between the S4-type voltage sensor and the pore: the S1-pore interface and the S4–S5 linker interface. (g) Comparison of current relaxation kinetics in the presence of Na+, Cs+and DMA for WT (solid black lines) and R2Q+WT mutant channel in the presence of Cs+(solid red line). Normalized currents were elicited by a depolarizing voltage step from 0 to +200 mV in the presence of 1 mM cGMP. Figure 8: Voltage-dependent gating in WT CNGA1 channels and possible underlying molecular mechanisms. ( a ) Dependence of P o / P o_max on V for Rb + from tail currents in WT (black circles), R2Q+WT (red squares) and R2Q_WT (green triangles) channels. Data were fitted with a Boltzmann function as described in the Methods with C, V 1/2 and z equal to: 0.77±0.01, 21.6±1.6 and 0.74±0.03 for WT; 0.69±0.01, 17.1±1.6 and 0.72±0.03 for R2Q+WT mutant; 0.70±0.01, 16.4±4.6 and 0.73±0.08 for R2Q_WT mutant channels. I t / I t_max is an estimation of P o / P o_max . ( b ) The same as in a but for Cs + . C, V 1/2 and z are as follow: 0.53±0.01, 29.5±1.9 and 0.52±0.02 for WT; 0.21±0.01, 87.1±0.9 and 0.47±0.01 for R2Q+WT mutant; 0.29±0.01, 50.8±3.1 and 0.54±0.03 for R2Q_WT mutant channels. ( c ) Dependence of P o / P o_max on V in MA for the same mutant channels as in a . C, V 1/2 and z are as follow: 0.21±0.01, 83.6±1.7 and 0.51±0.02 for WT; 0.09±0.02, 94.9±1.6 and 0.52±0.02 for R2Q+WT mutant; 0.06±0.01, 106.1±1.8 and 0.51±0.02 for R2Q_WT mutant channels. ( d ) Sequence alignment between the voltage sensor of CNGA1 and the Kv1.2–Kv2.1 chimera. Arginine residues (R) in S4 are highlighted in blue. Highly conserved negatively charged residues in S2 forming the external negative cluster (E214) and internal negative cluster (E224) are shown in red. ( e ) A cartoon of CNGA1 voltage sensor based on the crystal structure of Kv1.2–2.1 (PDB ID 2R9R) where the negative aspartate in position 202 could be involved in a salt bridge with Arg272 stabilizing the activated state of the voltage sensor is shown. ( f ) Cartoon of a monomeric subunit of chimera Kv1.2–Kv2.1 and the pore region from the adjacent subunit showing two possible interfaces (indicated by the squares) between the S4-type voltage sensor and the pore: the S1-pore interface and the S4–S5 linker interface. ( g ) Comparison of current relaxation kinetics in the presence of Na + , Cs + and DMA for WT (solid black lines) and R2Q+WT mutant channel in the presence of Cs + (solid red line). Normalized currents were elicited by a depolarizing voltage step from 0 to +200 mV in the presence of 1 mM cGMP. Full size image When Arg272 is neutralized, the P o at voltages of ~0 mV decreases ( Fig. 8b,c ), and inspection of the crystal structures of voltage sensors in voltage-gated channels provide a possible explanation. Indeed, in the chimeric Kv1.2/2.1 (refs [39] , [40] ) and NavAb (ref. 7 ) voltage-gated channels, the R2 and R3 residues interact with a conserved cluster of negative charges ( Fig. 8d,e ), stabilising the activated state. Moreover, sequence alignment between the voltage sensor of CNGA1 and the Kv1.2–Kv2.1 chimera ( Fig. 8d ) reveals that a key negatively charged residue (Glu214) in S2 is conserved in CNGA1, suggesting that a salt bridge between Arg272 and possibly Arg275 could stabilize the open state ( Fig. 8e ). Therefore, when Arg272 in S4 is neutralized (R2Q), the closed state could be stabilised. Our results show that in the presence of small alkali cations such as Li + , Na + or K + , and to some extent Rb + , the neutralisation of positive charges in S4 does not modify channel gating. In contrast, the permeation of large cations, such as Cs + , MA and DMA, is modified when Arg272 in S4 is neutralized, suggesting the possibility that S4 is involved in the voltage gating of these cations. Inspection of the crystal structure of voltage-gated channels and the analysis of conformational changes in Shaker K + channels could identify a possible molecular mechanism. In Shaker K + channels, conformational changes occurring in the S4-type voltage sensor are coupled to the S6 helix through the S4–S5 linker ( Fig. 8f ), composed of an alpha helix [18] , [39] , [40] . In contrast, this linker is unlikely to form an alpha helix in CNG channels, suggesting an impaired coupling [41] . A second interface between the voltage sensor and the pore domain, formed by a contact between S1 and the pore helix near the extracellular surface ( Fig. 8e ), has been identified [38] , [39] , [42] . Given the flexibility of the CNGA1 selectivity filter [43] , we speculate that permeation of larger cations leads to a tighter interaction between S1 and the P-helix. Therefore, we propose that in CNG channels, the S4-type voltage sensor does not control 'bundle crossing' as in K + channels, but it acts from the 'outside,' possibly through an interface between S1 and the pore helix near the extracellular surface. At positive voltages, the open pore widens, allowing the permeation of larger cations such as Cs + , MA and DMA. In the presence of these larger permeating cations, the cGMP-activated current raises with a time constant of 0.2 and 0.4 ms in symmetrical Cs + and DMA, respectively, when V is stepped from 0 to +200 mV, whereas this time constant is usually <100 μs in the presence of Na + ( Fig. 8g ). These longer time constants could reflect the time necessary to widen the pore. Point mutations that loosen the attachment of the selectivity filter to its surrounding structure result in mutant channels with impaired gating [27] that also become voltage dependent [44] . Indeed, the mutant channel desensitises when Glu363 is neutralized [10] , [27] , a voltage- and time-dependent process that is stronger at negative potentials ( Supplementary Fig. S2 ). Desensitisation of the mutant channel E363A, similar to C-type inactivation, is associated with conformational rearrangements of the residues in the outer vestibule [10] , [27] . Therefore, the molecular mechanisms underlying the voltage-dependent gating in WT CNGA1 channels, which is described, and in desensitising mutant channels could be different to some extent. Native CNG channels in rods and cones operate between −35 and −70 mV [11] , [45] , and because Na + and K + are the permeating ions, neither the pore nor the standard voltage sensors are operating. In fact, CNG channels have evolved to be permeable to Na + and K + at negative voltages, a strict requirement for the operation of phototransduction. Therefore, evolution, through the substitution of two amino acids (YG) in the filter of K + channels and the local modification of the amino-acid sequence of the interface between the voltage-sensing domain and the pore, has transformed a member of the family of voltage-gated channels into a non-voltage-gated channel, but only for Na + and K + . As a consequence of this substitution, CNG channels have also lost selectivity, allowing the permeation of Ca 2+ ions [13] and having a major role in the sensory adaptation in both photoreceptors and olfactory sensory neurons [46] , [47] . Molecular biology The 690-amino-acid CNGA1 channel was cloned from bovine rods. All mutations were made using mutagenesis as previously described [26] , [27] , and point mutations were confirmed by sequencing. For heterologous expression, the channels were subcloned into the expression vector pGEM-HE, and after plasmid DNA linearization and transcription, the RNA was injected in X. laevis oocytes. For experiments with co-expression, monomer co-injections were performed at a ratio of 1:1. Oocytes preparation WT and mutant channel RNAs were injected into X. laevis oocytes. The oocytes were prepared and injected as previously [26] , [27] described, and maintained at 19 °C (from 1 to 5 days after injection) in a Barth solution supplemented with 50 μg ml −1 of gentamycin sulphate and containing the following (in mM): 88 NaCl, 1 KCl, 0.82 MgSO 4 , 0.33 Ca(NO 3 ) 2 , 0.41 CaCl 2 , 2.4 NaHCO 3 and 5 Tris–HCl (pH 7.4 buffered with NaOH). During experiments, oocytes were kept in a Ringer solution containing the following (in mM): 110 NaCl, 2.5 KCl, 1 CaCl 2 , 1.6 MgCl 2 and 10 HEPES-NaOH, (pH 7.4 buffered with NaOH). Rods isolation Using Cynops ensicauda newts as previously described [48] , isolated rods or detached rod outer segments were obtained by repeatedly dipping small pieces of retina into a Sylgard Petri dish with a Ringer solution containing the following (in mM): 110 NaCl, 2.5. KCl, 1 CaCl 2 , 1.6 MgCl 2 , and 3 HEPES-NaOH, 0.01 EDTA and 10 Glucose (pH 7.7–7.8 buffered with NaOH). All the studies carried out using X. laevis and C. ensicauda have been approved by the SISSA's Ethics Committee according to the Italian and European guidelines for animal care (d.l. 116/92; 86/609/C.E.). Electrophysiology and solutions cGMP-gated currents from recombinant WT and CNGA1 mutant channels were excised from oocytes, and cGMP-gated currents from native CNG channels were excised from rod outer segments as previously described [13] , [26] . cGMP-gated currents evoked by 1 mM cGMP from excised patches were recorded under voltage-clamp conditions. Borosilicate glass electrode resistance was ~2–5 MΩ for an excised patch on an oocyte membrane and 10–20 MΩ for an excised patch on rod. Solutions on both sides of the membrane consisted of the following (in mM): 110 XCl, 10 HEPES and 0.2 EDTA (pH 7.4), where X is the indicated alkali or organic cation. Voltage control and current acquisition were achieved with a Digidata 1322A (Molecular Devices) board, an Axopatch 200 patch clamp (Molecular Devices) and Clampex Software (Molecular Devices). Different voltage step protocols were used for different recordings (see figure legends). Data are usually given as the means±s.e.m., and n corresponds to the number of experiments. Salts and reagents were purchased from Sigma. The dependence of P o / P o_max on V was fitted by a Boltzmann equation plus a pedestal (C): where the pedestal (C) indicates the existence of a closed to open transition independent of voltage, k is the slope factor and V 1/2 is the activation midpoint of the voltage-dependent component. The effective charge ( z ) can be obtained using z = RT / kF , where T =295 K, and R and F are the gas and the Faraday constants, respectively. Noise analysis In the presence of 1 mM cGMP, WT CNGA1 channels have a dominant single-channel conductance ( γ sc ) [33] , [34] . Under these conditions, the noise variance ( σ I 2 ) is related to the amplitude of the mean current ( I ) by the following equation: where i sc is the amplitude of the single-channel current and n is the number of channels present in the membrane patch [49] . Hence, the ratio σ I 2 / I of the variance of current fluctuations ( σ I 2 ) and of the mean current ( I ) is the following: where P o is the single-channel open probability. This ratio is independent from the number of channels present in the membrane patch and is expected to increase when i sc increases and/or P o decreases. When P o becomes negligible (that is, at low cGMP concentrations), σ I 2 / I approximates i sc , allowing an estimation of single-channel conductance from the macroscopic current fluctuation analysis. Single-channel analysis Single-channel currents ( i sc ) were determined from all-point amplitude histograms of current fluctuations in the presence of 1 mM cGMP. Histograms were normalized so that their area was equal to 1 and were fitted as the sum of two or three Gaussian functions using a Levenberg–Marquardt least-squares minimization method (pClamp 10.1) to provide the values of i sc (ref. 20 ). Rapid flickering openings observed in the WT channel at −160 mV for Cs + and in other mutant channels do not allow for a reliable evaluation of i sc from the all-point amplitude histograms, and i sc was measured from single fluctuation peak currents [50] . Only transitions lasting at least 2 filter rise times were considered, allowing the current to reach at least 98.8% of its true amplitude [51] , [52] during channel openings. Histograms obtained from the peak current analysis procedure were fitted with a Gaussian distribution, providing the corresponding estimation of single-channel amplitude ( i sc_p ). Open probabilities ( P o ) were estimated from the all-point amplitude histograms obtained from patches containing only one CNGA1 channel as 1- P c . Closed probability ( P c ) was determined from the area of the Gaussian component associated to the closed state of the channel. Molecular modelling Sequence alignments were based on published data [25] , [29] ( Figs 3a and 6a ) or performed using ClustalW [53] ( Fig. 8d ). Cartoons were prepared using known structures of K v and NaK chimeric channels available in the Protein Data Bank (PDB) using the DeepView module of the Swiss-PDBViewer (v4.04) and VMD (v1.8.7) software [54] , [55] . How to cite this article: Marchesi, A. et al . Gating of cyclic nucleotide-gated channels is voltage dependent. Nat. Commun. 3:973 doi: 10.1038/ncomms1972 (2012).